A unified strategy toward total syntheses of lindenane sesquiterpenoid [4 + 2] dimers 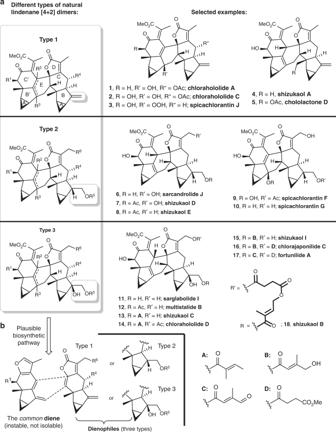Fig. 1 Three types of natural lindenane [4 + 2] dimers and related biosynthetic hypothesis.aThe dimeric lindenane sesquiterpenoids can be categorized into three types, among which type 3 dimers are superior in numbers.bThe skeleton of the dimeric lindenane sesquiterpenoids can be constructed through a [4 + 2] cycloaddition between the common diene and different types of dienophiles The dimeric lindenane sesquiterpenoids are mainly isolated from the plants of Chloranthaceae family. Structurally, they have a crowded molecular scaffold decorated with more than 11 stereogenic centers. Here we report divergent syntheses of eight dimeric lindenane sesquiterpenoids, shizukaols A, C, D, I, chlorajaponilide C, multistalide B, sarcandrolide J and sarglabolide I. In particular, we present a unified dimerization strategy utilizing a base-mediated thermal [4 + 2] cycloaddition between a common furyl diene, generated in situ, and various types of dienophiles. Accordingly, all the three types of lindenane [4 + 2] dimers with versatile biological activities are accessible, which would stimulate future probing of their pharmaceutical potential. The dimeric lindenane sesquiterpenoids are a group of biologically active complex natural products mainly isolated from the plants of Chloranthaceae family. Structurally, these [4 + 2] dimers possess congested frameworks of at least eight rings decorated by more than 11 stereogenic centers [1] , [2] , [3] . Three types (types 1–3, Fig. 1a ) can be categorized according to various substitution pattern on the ring B. Owing to their structural diversity and biological activities, numerous efforts have been made toward syntheses of the corresponding dimers or monomers [4] , [5] , [6] , [7] , [8] , [9] , [10] , [11] , [12] , [13] , [14] , [15] , [16] , [17] , [18] , [19] , [20] , [21] . Following our long-standing interest in the syntheses of terpenoids [22] , we reported the first syntheses of lindenane sesquiterpenoid [4 + 2] dimers, sarcandrolide J and shizukaol D (type 2) in the guidance of our modified biosynthetic hypothesis (Fig. 1b ) [6] . Recently, the Peng group reported their achievement of total syntheses of shizukaols A and E, types 1 and 2 [4 + 2] dimers, respectively, through the other modified biomimetic Diels–Alder reaction [7] . Fig. 1 Three types of natural lindenane [4 + 2] dimers and related biosynthetic hypothesis. a The dimeric lindenane sesquiterpenoids can be categorized into three types, among which type 3 dimers are superior in numbers. b The skeleton of the dimeric lindenane sesquiterpenoids can be constructed through a [4 + 2] cycloaddition between the common diene and different types of dienophiles Full size image However, no synthesis of type 3 [4 + 2] dimers has yet been reported, despite their predominant numbers accounting for more than four-fifths across the whole lindenane family. Notably, direct functionalization of the gem -disubstituted alkene on ring B failed to convert type 1 dimers into types 2 or type 3, because the inherent stereochemical control from the robust 3/5/6/5 backbone favors the undesired diastereomer [6] , [16] . Thus, a unified synthetic strategy is in demand to provide all the three types of lindenane [4 + 2] dimers and their synthetic analogs, by following the plausible [4 + 2] biosynthetic pathways with a common furyl diene and various dienophiles. Since the corresponding furyl diene is instable and not isolable, an acid-mediated diene-formation is pivotal to trigger the subsequent cycloaddition in our previous synthesis of type 2 [4 + 2] dimers (Fig. 2a ) [6] . However, the gem -disubstituted alkene substructure on ring B of type 1 dimers may be vulnerable under acidic conditions, as the acid-promoted exo/endo cyclic alkene isomerization was observed, transforming bolivianine to isobolivianine (Fig. 2b ) [23] , [24] , [25] . Fig. 2 Evolution from an acid-promoted cascade to the current unified strategy. a The skeleton of type 2 dimeric lindenane sesquiterpenoids was constructed through an acid-promoted diene-formation/[4 + 2] cascade. b Bolivianine was transformed to isobolivianine via the acid-promoted exo / endo cyclic alkene isomerization. c A unified synthetic strategy is developed for the synthesis of three types of dimeric lindenane sesquiterpenoids Full size image We conceive and realize a unified base-promoted strategy enabling divergent and biomimetic syntheses of all types of lindenane [4 + 2] dimers (Fig. 2c ). Among this strategy, a type 3 lindenane dimer, sarglabolide I, could serve as a common synthetic precursor toward other type 3 dimers through versatile acetylations. Of note, the common diene precursor used in this strategy is more synthetically viable than that previously used in acid-promoted cycloaddition (12 steps vs. 17 steps). Synthesis of the diene precursor We initiated synthesis of the common diene precursor from a known Michael adduct 19 from verbenone (Fig. 3a ) [23] , [24] , [25] . Oxidation to a 1,2-diketone and subsequent ring-opening of the cyclobutane in the presence of boron trifluoride afforded enone 20 . Then, a formal oxidative [3 + 2] cycloaddition in the presence of cerium ammonium nitrate (CAN), followed by treatment with Amberlsyt-15, was employed between compound 20 and silyl enol ether 21a to afford adduct 22 [26] , [27] . Other single oxidants such as 2,3-Dichloro-5,6-dicyano- p -benzoquinone (DDQ) and Cerium(IV) sulfate only got the complex mixture. Intriguingly, acetonitrile/benzene (4:1) co-solvents serve as the optimal solvent system for the oxidative coupling step, whereas the individual solvent only delivered inferior results, probably due to compromised equilibrium between solubility of CAN and the solvent polarity. Moreover, application of 21b and 21c instead of 21a in this reaction resulted in lower yields. Mechanistically, CAN may serve as the single electron oxidant to convert 21a into the radical cation I , which could undergo a radical Michael addition to compound 20 [26] . The forming intermediate II would be further oxidized to the cationic intermediate III , which would be quenched by water to produce a mixture of aldehyde IVa and semi-acetal IVb . Subsequently, Amberlyst-15 promoted dehydration and facilitated aromatization to give furan 22 (Fig. 3b ). Fig. 3 Synthesis of the diene precursor 25 . a Compound 25 can be synthesized from compound 19 in 11 steps. b The mechanism for formation of 22 was proposed. DCM = dichloromethane, DMF = N,N -dimethylformamide, Ac = acetyl, DIPEA = N,N -diisopropylethylamine, MOMCl = methoxymethyl chloride Full size image A chemo-selective allylic oxidation of 22 yielded an enal smoothly using selenium dioxide, while the furyl methylene and methyl remained untouched. The hydrazone formation followed by the Rh-catalyzed intramolecular cyclopropanation generated compound 23 with proper stereochemistry. In contrast, our original Pd-catalyzed cyclopropanation was proved unsuccessful [28] . Treating 23 with SeO 2 yielded 24 and an unidentified intermediate presumably as allylic selenide [29] , [30] , [31] . Accordingly, sodium periodate was introduced into the reaction mixture, exclusively producing 24 in 83% yield [32] , [33] , [34] , while no furan benzylic oxidation product was detected. Finally, acid-promoted acetylation of the tertiary alcohol, diastereoselective reduction of the ketone, and the MOM protection resulted in diene precursor 25 . Mesylation and tosylation of the corresponding tertiary alcohol of compound 24 failed due to low reactivity. Synthesis of the dienophile We validated our proposed unified synthetic strategy by first aiming at total syntheses of type 3 [4 + 2] dimers. Thus, sarglabolide I ( 11 ) was chosen as the first target molecule and we began to synthesize the corresponding dienophile partner 36 for sarglabolide I ( 11 ) from the known compound 26 (Fig. 4a ), accessible from verbenone [6] , [23] , [24] , [25] . Fig. 4 Synthesis of the dienophile 36 for type 3 [4 + 2] natural dimers. a Compound 36 can be synthesized from 26 in 8 steps. 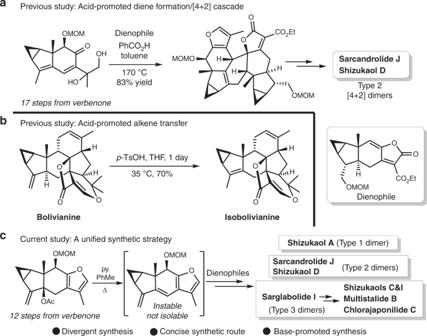Fig. 2 Evolution from an acid-promoted cascade to the current unified strategy.aThe skeleton of type 2 dimeric lindenane sesquiterpenoids was constructed through an acid-promoted diene-formation/[4 + 2] cascade.bBolivianine was transformed to isobolivianine via the acid-promotedexo/endocyclic alkene isomerization.cA unified synthetic strategy is developed for the synthesis of three types of dimeric lindenane sesquiterpenoids b Direct dihydroxylation of 26 fails to afford the desired diol 27 . c Both Prévost trans -dihydroxylation and sequential halogen hydroxylation-basic hydrolysis fail to afford 27 . PPTS = pyridinium p -toluenesulfonate Full size image Direct dihydroxylation of 26 failed to afford the desired diol 27 using either K 2 OsO 4 •2H 2 O/NMO or Sharpless asymmetric dihydroxylation (SAD) with both AD-mix-α and AD-mix-β. Instead, while compound epi- 27 was obtained as the major diastereomer with more than 20:1 dr in all cases (Fig. 4b ). We rationalize that these results should come from intrinsic stereochemical control of the rigid chiral skeleton of 26 . Thus, we subjected 26 to both Prévost trans- dihydroxylation and sequential halogen hydroxylation-basic hydrolysis, attempting to hydrolyze epoxide 30 to deliver 27 . Compound 30 could be presumably formed through capture of the cyclic halonium ion 28 by hydroxide or carboxylate and subsequent epoxidation from 29 (path a, Fig. 4c ). However, only allylic halogen, allylic alcohol and allylic acetate were formed instead, indicating that the undesired base-promoted deprotonation of 28 proceeded faster to give 31 , transformable to other allylic compounds (path b, Fig. 4c ). Thus, we resorted to an alternative route. Ozonolysis of 26 , followed by a cautious workup without adding any reductant, resulted in ketone 32 with minimal epimerization of C5. Although Julia olefination of 32 was feasible to give 26 [10] , [15] , reacting 26 with MOMOCH 2 SnBu 3 / n BuLi at either −78 °C or 0 °C only led to isomerization at C5 to give 33 , serving as a thermodynamic sink with stabilized cis -fused 5/6-bicycle. So we considered application of less bulky vinyl organometallic reagent to increase rate of the nucleophilicity over basic isomerization at C5. While vinyl Grignard reagent failed to provide 34 in significant yield, the corresponding cerium reagent afforded 33 as the only byproduct, although organocerium reagents feature high nucleophilicity and weak basicity [35] , [36] . Fortunately, vinyl lithium promoted the reaction at −78 °C to give 33 and the desired adduct 34 in 34% and 39% yield, respectively. Pleasingly, after several trials, we found the desired nucleophilic reaction would surpass the undesired enolization of 32 much more at higher temperature. In this manner, vinyl lithium was manifested to generate 34 in 61% yield at −10 °C. Ozonolysis of 34 followed by an in situ reduction successfully afforded diol 27 . It was further protected as an acetonide and the glycol-protected ketal was removed under acidic conditions to give compound 35 , which was transformed to 36 over three steps. Total syntheses of type 3 [4 + 2] lindenane dimers With both 25 and 36 in hand, we next executed the diene-formation/cycloaddition cascade. As shown in Fig. 5 , diene precursor 25 was pre-mixed with dienophile 36 and pyridine in a sealed tube upon the heat. The extrusion of acetate generated diene 37 in situ, which underwent an intermolecular [4 + 2] cycloaddition with 36 to form cycloadduct 39 as the major diastereomer. An optimal 71% yield of 39 was obtained at 200 °C, whereas a Cope rearrangement byproduct ( 38 ) was also observed, which is stable under this thermal condition. After simultaneous deprotection of MOM ether and acetonide and reduction of the ethyl ester, compound 40 was obtained in 75% yield over two steps. A one-pot protocol afforded sarglabolide I ( 11 ) in 87% yield through sequential photolytic oxidation of the furan and esterification of the resultant acid [37] . Selective esterifications of 11 using acetic anhydride and tiglic acid afforded multistalide B ( 12 ) and shizukaol C ( 13 ), respectively [38] , [39] . Shizukaol C exhibits potent inhibitory activities against various plant pathogenic fungi [40] . In addition, acylation of sarglabolide I ( 11 ) offered compound 43 utilizing acid 41 , and the final silyl deprotection afford shizukaol I ( 15 ) [41] . 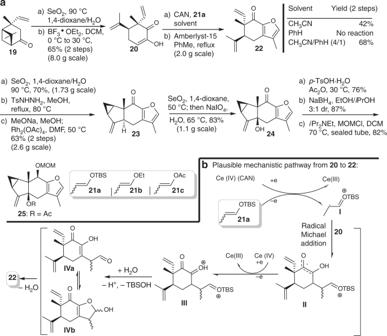Fig. 3 Synthesis of the diene precursor25.aCompound25can be synthesized from compound19in 11 steps.bThe mechanism for formation of22was proposed. DCM = dichloromethane, DMF =N,N-dimethylformamide, Ac = acetyl, DIPEA =N,N-diisopropylethylamine, MOMCl = methoxymethyl chloride Moreover, the second O- acylation of 43 gave compound 44 , which went through silyl deprotection to afford chlorajaponilide C ( 16 ) [42] , [43] . 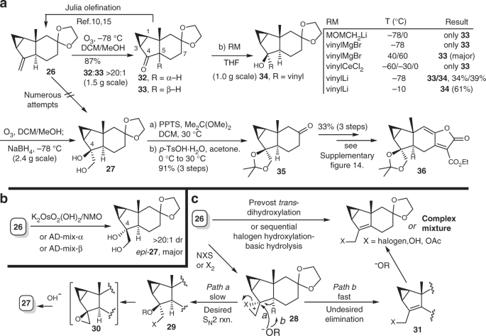Fig. 4 Synthesis of the dienophile36for type 3 [4 + 2] natural dimers.aCompound36can be synthesized from26in 8 steps.bDirect dihydroxylation of26fails to afford the desired diol27.cBoth Prévosttrans-dihydroxylation and sequential halogen hydroxylation-basic hydrolysis fail to afford27. PPTS = pyridiniump-toluenesulfonate Notably, this natural product shows very potent Plasmodium falciparum growth inhibition with IC 50 as low as 1.1 nM; it was further tested for mammalian cytotoxicity with WI-38 cell line and show selective index as high as 4900 [43] . These findings indicate impressive potential as anti-malarial drug for this compound. Fig. 5 Total syntheses of type 3 [4 + 2] lindenane dimers. TPP = 5,10,15,20-tetraphenylporphyrin, DMAP = N,N -4-dimethylaminopyridine, EDCI = 1-ethyl-3-(3-dimethylaminopropyl)carbodiimide hydrochloride, MNBA = 2-methyl-6-nitrobenzoic anhydride Full size image Total syntheses of [4 + 2] lindenane dimers of types 1 and 2 We further applied the unified strategy in synthesis of type 1 and type 2 dimers (Fig. 6a ). In the presence of pyridine, mixing compound 25 and previously reported dienophile 45 [6] , generated compound 46 as the major diastereomer ( > 20:1 dr) under thermal conditions. In accordance with reported protocols [6] , 46 can be transformed into sarcandrolide J ( 6 ) and shizukaol D ( 7 ), two [4 + 2] lindenane dimers of type 2 [44] , [45] , [46] , [47] . Similarly, compound 48 was synthesized in a moderate yield (43%) by heating the mixture of 25 and chloranthalactone A ( 47 ), synthesized from verbenone as well [17] , [18] , [23] , [24] , [25] . After deprotection of the MOM ether and oxidative elaboration of the furan ring, shizukaol A ( 4 ), a [4 + 2] lindenane dimer of type 1 [48] , was synthesized. In comparison with the 16% yield of 48 acquired from the acid-mediated dimerization between 47 and previously known 49 (Fig. 6b ) [6] , this base-mediated dimerization protocol showcases its satisfactory synthetic efficacy and panoramic tolerance of versatile dienophiles. Fig. 6 Total syntheses of [4 + 2] lindenane dimers of types 1 and 2. a Sarcandrolide J, shizukaol D and shizukaol A can be synthesized through the [4 + 2] cycloaddition promoted by base. b The acid-mediated cycloaddition between 47 and 49 afforded 48 in inferior yield to that of the base-mediated cycloaddition between 25 and 47 Full size image In summary, we developed an effective and unified strategy enabling feasible access to all the three types of lindenane sesquiterpenoid [4 + 2] dimers exemplified by syntheses of eight natural products. This natural family composes of more than one hundred dimeric compounds possessing versatile biological activities. Our divergent strategy would undoubtedly lay solid foundation for creation of the analog library and thus facilitate biological evaluations of these lindenane dimers. General All reactions were performed under an argon atmosphere with dry solvents under anhydrous conditions, unless otherwise stated. DCM, DIPA, DIPEA, HMDS, MeCN, DMF, Et 3 N, and toluene were distilled from calcium hydride under argon; MeOH was distilled from dry magnesium turnings and iodine under argon; THF was distilled from sodium-benzophenone under argon; Ac 2 O was distilled from K 2 CO 3 after being preprocessed by P 2 O 5 . Unless otherwise noted, all the other chemicals were purchased commercially and used without further purification. Flash chromatography was performed using silica gel (200–300 mesh). 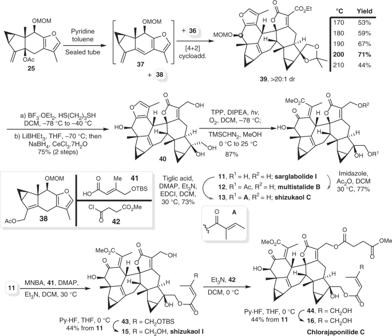Fig. 5 Total syntheses of type 3 [4 + 2] lindenane dimers. TPP = 5,10,15,20-tetraphenylporphyrin, DMAP =N,N-4-dimethylaminopyridine, EDCI = 1-ethyl-3-(3-dimethylaminopropyl)carbodiimide hydrochloride, MNBA = 2-methyl-6-nitrobenzoic anhydride 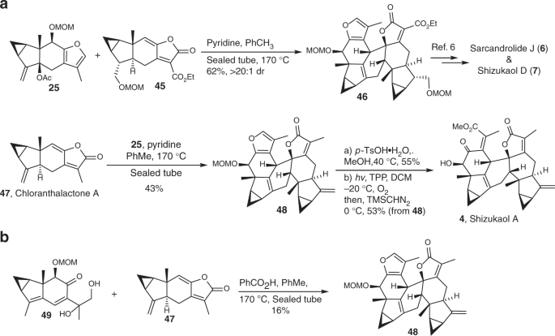Fig. 6 Total syntheses of [4 + 2] lindenane dimers of types 1 and 2.aSarcandrolide J, shizukaol D and shizukaol A can be synthesized through the [4 + 2] cycloaddition promoted by base.bThe acid-mediated cycloaddition between47and49afforded48in inferior yield to that of the base-mediated cycloaddition between25and47 Thin layer chromatography (TLC) was used for monitoring reactions and visualized by a UV lamp (254 nm and 365 nm), I 2 and developing the plates with p -anisaldehyde or phosphomolybdic acid. 1 H and 13 C NMR were recorded on Bruker DRX-400 MHz NMR spectrometer or Bruker 800 MHz NMR spectrometer with TMS as the internal standard and were calibrated using residual undeuterated solvent as an internal reference (CDCl 3 : 1 H NMR = 7.26, 13 C NMR = 77.16; C 6 D 6 : 1 H NMR = 7.16, 13 C NMR = 128.06; CD 3 COCD 3 : 1 H NMR = 2.05, 13 C NMR = 29.84; CD 3 OD: 1 H NMR = 3.31 and 4.87, 13 C NMR = 49.00; Pyridine-d 5 : 1 H NMR = 8.74, 7.58 and 7.22). Abbreviations in 1 H NMR data are illustrated as follows: s = singlet, d = doublet, t = triplet, dd = doublet of doublet, ddd = doublet of doublet of doublet, dt = doublet of triplet, td = triplet of doublet, m = multiplet, br = broad. Coupling constants ( J ) are reported in Hertz (Hz). Optical rotations were measured at the sodium D line with a 100 mm path length cell, and are reported as follows: [α] D T , concentration (g/100 mL), and solvent. High-resolution mass spectra (HRMS) were recorded by using Bruker-FT-MS spectrometers. Infrared (IR) spectra were recorded on a NEXUS 670 FT-IR device and are reported in wavenumbers (cm −1 ). Experimental data For detailed experimental procedures, see Supplementary Methods. For NMR spectra of the synthesized compounds in this article, see Supplementary Figs. 26 – 94 . For the comparison of NMR spectra of the natural products and synthetic products, see Supplementary Tables 1 – 12 .